Stretching fibronectin fibres disrupts binding of bacterial adhesins by physically destroying an epitope Although soluble inhibitors are frequently used to block cell binding to the extracellular matrix (ECM), mechanical stretching of a protein fibre alone can physically destroy a cell-binding site. Here, we show using binding assays and steered molecular dynamics that mechanical tension along fibronectin (Fn) fibres causes a structural mismatch between Fn-binding proteins from Streptococcus dysgalactiae and Staphylococcus aureus. Both adhesins target a multimodular site on Fn that is switched to low affinity by stretching the intermodular distances on Fn. Heparin reduces binding but does not eliminate mechanosensitivity. These adhesins might thus preferentially bind to sites at which ECM fibres are cleaved, such as wounds or inflamed tissues. The mechanical switch described here operates differently from the catch bond mechanism that Escherichia coli uses to adhere to surfaces under fluid flow. Demonstrating the existence of a mechanosensitive cell-binding site provides a new perspective on how the mechanobiology of ECM might regulate bacterial and cell-binding events, virulence and the course of infection. Despite the intensive research on bacterial adhesins, so far there is no evidence that mechanical factors might regulate the binding efficiency of bacterial adhesins to extracellular matrix (ECM). Pathogens often begin host invasion by binding to ECM proteins, which display a variety of specific adhesion sites for bacteria and eukaryotic cells. Numerous microbes have evolved cell-surface proteins that expose recognition sequences for a majority of host ECM proteins, including fibronectin (Fn) [1] and serum proteins [2] , [3] , leading to a wide variety of diseases, including wound infections. Fn is a glycoprotein that circulates in body fluids (300 μg ml −1 ) as a soluble compact dimer and is assembled by cells into insoluble ECM fibres [4] , [5] . It has a critical role in wound healing, in which its expression and fibrillogenesis are known to be upregulated to assist tissue regeneration [6] , [7] , thus making it a well-suited target for bacterial binding [8] . Many bacteria, including Staphylococcal, Streptococcal strains and Spirochetes, express cell-wall-anchored Fn-binding proteins (FnBP) that recognize the same binding site on Fn [9] , [10] . The multimodularity of Fn ( Fig. 1a ) allows spatial distribution of distinct recognition sites along the molecule, enabling diverse interactions such as with other ECM proteins, growth factors, and prokaryotic and eukaryotic cells [11] . Dimeric Fn contains more than 50 modules that belong to one of the three structural β-sheet motifs, FnI, FnII and FnIII [12] . To enhance specificity, the bacterial FnBP exploits the modular structure of Fn by simultaneously binding to several FnI modules that define the amino (N)-terminal 29 KDa region [13] , [14] ( Fig. 1b ). The bacterial FnBP aligns antiparallel with up to five FnI modules and undergoes a disordered–ordered transition upon binding to form a tandem β-zipper [15] . A comparison of FnBP across different classes of bacteria shows that the bacterial Fn-binding repeats (FnBR) are each made up of 35–40 residues that form the primary binding site to Fn, but the number of FnBR varies considerably across species, containing just one for Borrelia burgdorferi [16] and 11 for Staphylococcus aureus [17] ( Fig. 1b ). The significance of this variation in relation to the specific modes of host adhesion and invasion is not known. 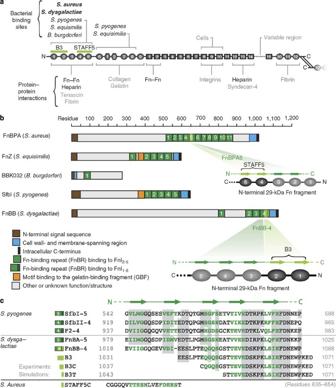Figure 1: Structural organization of Fn and the bacterial FnBP. (a) Schematic representation of the multimodular structure of Fn emphasizing specific binding sites for cells and matrix proteins. The Fn modules type I, II and III are represented as circles, hexagons and rectangles, respectively. (b) Domain organization of five FnBP from various bacteria, including the peptides used in this study: B3 from FnBB-4 ofS. dysgalactiaeand STAFF5 from FnBPA5 ofS. aureus. (c) Sequence alignment of various FnBR binding to FnI1–5fromS. pyogenesandS. dysgalactiae(alignment as shown in ref.56). Grey regions indicate conserved residues; letters in green are the residues mainly involved in β-sheet interactions with the corresponding Fn modules; and the numbers correspond to the first and last residues. For site-specific photolabelling, the B3 moiety was synthesized with an additional N-terminal cysteine (B3C). B3T, the truncated form of the B3 peptide, is part of the nuclear magnetic resonance structure that has been used for SMD simulations (PDB-code 1O9A). The sequence of peptide STAFF5C is given in the last line. Figure 1: Structural organization of Fn and the bacterial FnBP. ( a ) Schematic representation of the multimodular structure of Fn emphasizing specific binding sites for cells and matrix proteins. The Fn modules type I, II and III are represented as circles, hexagons and rectangles, respectively. ( b ) Domain organization of five FnBP from various bacteria, including the peptides used in this study: B3 from FnBB-4 of S. dysgalactiae and STAFF5 from FnBPA5 of S. aureus . ( c ) Sequence alignment of various FnBR binding to FnI 1–5 from S. pyogenes and S. dysgalactiae (alignment as shown in ref. 56 ). Grey regions indicate conserved residues; letters in green are the residues mainly involved in β-sheet interactions with the corresponding Fn modules; and the numbers correspond to the first and last residues. For site-specific photolabelling, the B3 moiety was synthesized with an additional N-terminal cysteine (B3C). B3T, the truncated form of the B3 peptide, is part of the nuclear magnetic resonance structure that has been used for SMD simulations (PDB-code 1O9A). The sequence of peptide STAFF5C is given in the last line. Full size image In wounds, bacteria encounter both soluble plasma Fn and fibrillar matrix Fn [18] , [19] . Although the interaction of bacterial FnBP with either surface adsorbed Fn or Fn in solution is well characterized [17] , [20] , it is not known whether tensile mechanical forces might have a role in regulating the interaction of bacterial adhesins with ECM molecules. Fn in fibrillar matrix is known to have distinctly different conformations compared with soluble Fn or surface-adsorbed dimeric Fn (as reviewed in ref. 11 ). Cells assemble Fn into matrix fibres [21] , [22] , and cell-generated forces are sufficient to stretch and partially unfold fibrillar Fn [23] , [24] , thus stabilizing a broad range of new conformations that are not found under equilibrium conditions. Significant in the context of understanding Fn as a mechanoregulated protein were the findings that the stretching of Fn fibres can disrupt an antibody epitope located between FnI 9 and FnIII 1 (ref. 25 ) and expose cryptic binding sites in FnIII modules that are buried in relaxed Fn fibres [26] . How does mechanoregulation of fibrillar Fn impact specific Fn-mediated bacterial adhesion? The heterogeneous distribution of Fn molecular conformation in the ECM of living cells [23] , [24] makes it difficult to directly show bacterial binding being affected by ECM fibre tension, as the size of bacteria is at the typical length scale at which stretch-induced structural heterogeneities exist in native ECM. To circumvent this problem, here we use a cell-free binding assay that allows the stretching of single Fn fibres through the full range of physiologically relevant conformations that are present in cell culture [25] , [27] . To explore whether tensile forces exerting an effect on protein fibres can regulate the binding of an adhesin, a bacterial peptide that is part of an FnBR from Streptococcus dysgalactiae , was used as a high-resolution structure in complex with the fragment FnI 1-2 is available [15] . S. dysgalactiae , the causative agent for bovine mastitis [28] , has four FnBRs that can potentially interact with not just one but multiple Fn molecules within a fibril. The FnBP-containing adhesins expressed on the bacterial surface are up to 1,000 amino-acids long and contain potentially other specific and nonspecific binding sites that could interact with Fn or other ECM components [10] . Here, we explore how the specific binding of two short bacterial peptides B3 and STAFF5, derived from S. dysgalactiae and S. aureus , respectively, are modulated by stretching Fn fibres ( Fig. 1b,c ). To understand the underlying structural aspects of mechanoregulation, we used steered molecular dynamic (SMD) simulations to determine how tensile force applied to the B3T–FnI 1-2 complex could alter the hydrogen-bond network defining this receptor–ligand interaction. Together with the experimental results derived from the Fn-binding assay, we show that both bacterial peptides bind significantly less to stretched than to relaxed Fn fibres, thus demonstrating the mechanoregulation of a cell-binding site on the N-terminus of Fn. Stretching Fn fibres destroys the bacterial binding site To determine whether mechanical strain alters the binding of a bacterial adhesin, a fragment B3 of FnBR-4 from S. dysgalactiae ( Fig. 1b ) was used. The B3 peptide ( Fig. 1c ) was synthesized with an additional N-terminal cysteine residue (B3C) in order to label it with Alexa Flour-488 dye (B3C-488). A binding assay that allows the stretching of single Fn fibres through the full range of physiologically relevant conformations (from fully relaxed to breakage) [27] was used in combination with optical colocalization studies to experimentally verify strain-dependent binding [25] . Fn fibres were manually deposited on stretchable silicone sheets ( Fig. 2a,b ). To quantify the binding, ratiometric measurements of labelled B3C-488 bound to Fn fibres that contained Cy5-labelled Fn were observed as a function of fibre extension (mechanical strain; Fig. 2c ). Depositing fibres in different orientations on the same sheet allowed an overview of differential binding as a function of strain. To increase statistical significance, we deposited fibres parallel to each other that are under the same mechanical strain ( Fig. 3a–f ). The intensity ratio of the labelled B3C-488 (I B3C-488 ) per labelled Fn (I Fn-Cy5 ) versus the mechanical strain shows that the binding of the bacterial peptide B3C-488 decreased significantly when fibres were stretched ( Fig. 4a ). 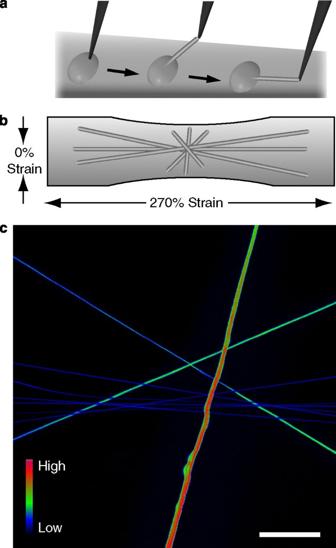Figure 2: Fn fibre stretch assay to quantify mechanosensitive bacterial peptide binding. (a) Fn fibres were made by dipping a sharp tip into a drop of PBS containing 0.5 g l−1Fn (5% Fn-Cy5 and 95% unlabelled Fn), which is then gently pulled back to induce Fn polymerization into fibres. (b) These prestrained fibres are subsequently deposited onto stretchable silicone sheets27in various orientations to the horizontal strain axis, resulting in variable degrees of fibre strains. (c) Confocal micrograph depicting fluorescent intensity ratios of bacterial peptide B3C-488 binding to Fn-Cy5 fibres, shown here in false colours. Scale bar: 50 μm. Figure 2: Fn fibre stretch assay to quantify mechanosensitive bacterial peptide binding. ( a ) Fn fibres were made by dipping a sharp tip into a drop of PBS containing 0.5 g l −1 Fn (5% Fn-Cy5 and 95% unlabelled Fn), which is then gently pulled back to induce Fn polymerization into fibres. ( b ) These prestrained fibres are subsequently deposited onto stretchable silicone sheets [27] in various orientations to the horizontal strain axis, resulting in variable degrees of fibre strains. ( c ) Confocal micrograph depicting fluorescent intensity ratios of bacterial peptide B3C-488 binding to Fn-Cy5 fibres, shown here in false colours. Scale bar: 50 μm. 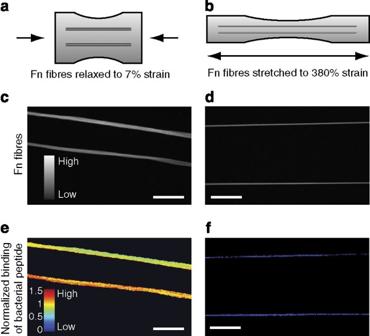Figure 3: Binding of photolabelled bacterial peptide B3C to Fn fibres. Schematic representation of Fn fibres (a) relaxed and (b) stretched on elastic silicone substrates manipulated using a uniaxial mechanical straining device26. Confocal micrographs depicting fluorescence intensity values of (c) relaxed and (d) stretched Fn fibres. Corresponding confocal images of the same fibres as shown incandd, indicating the normalized intensity ratios of B3C-488 versus Fn-Cy5 in false colours for (e) relaxed and (f) stretched Fn fibres. Fibres were deposited in parallel arrangements to increase the sample size for each strain value. Scale bar: 50 μm. Full size image Figure 3: Binding of photolabelled bacterial peptide B3C to Fn fibres. Schematic representation of Fn fibres ( a ) relaxed and ( b ) stretched on elastic silicone substrates manipulated using a uniaxial mechanical straining device [26] . Confocal micrographs depicting fluorescence intensity values of ( c ) relaxed and ( d ) stretched Fn fibres. Corresponding confocal images of the same fibres as shown in c and d , indicating the normalized intensity ratios of B3C-488 versus Fn-Cy5 in false colours for ( e ) relaxed and ( f ) stretched Fn fibres. Fibres were deposited in parallel arrangements to increase the sample size for each strain value. Scale bar: 50 μm. 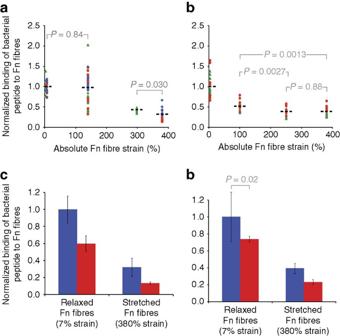Figure 4: Experimental validation of mechanosensitive binding of bacterial peptides to Fn fibres. (a,b) Strain-dependent binding of bacterial peptides B3C-Alexa488 and STAFF5C-Alexa488 to Cy5-labelled Fn fibres. The mean of the intensity ratios (IB3C-488/IFn-Cy5) of relaxed fibres was set to 1 and the other values were scaled accordingly. All mean values (shown by black bar) are significantly different from each other withP<0.001 (unpaired two-tailed Student'st-test), except where noted. (a) Intensity ratio plot of Alexa488-labelled B3C to Cy5-labelled Fn fibres versus Fn fibre strain (see Fig. 3). Each experiment (shown as differently shaped and coloured data points) consisted of 30 fibres: 10 were relaxed (∼7% strain), 10 deposited only in a prestrained state (no mechanical manipulation of the silicone sheet,∼140% strain26) and 10 stretched (∼300 or∼380% strain). (b) Intensity ratio plot of Alexa488-labelled STAFF5C to Cy5-labelled Fn fibres versus Fn fibre strain. Each experiment (shown as differently shaped and coloured data points) consisted of 40 fibres, including 20 relaxed (∼0 and∼100% strain) and 20 stretched fibres (∼250 and∼380% strain). Inhibition of strain-dependent binding of the bacterial peptide B3C-Alexa488 to Cy5-labelled Fn fibres in the presence (red bars) of (c) soluble Fn (300 μl mg−1) and (d) heparin (100 μl mg−1). The mean of the intensity ratio of relaxed fibres in the absence (blue bars) of soluble Fn or heparin was set to 1 and the remaining three values were scaled accordingly. All values are significantly different from each other (unpaired two-tailed Student'st-test) withP<0.0001, except where indicated. Values are means of intensity ratios of 20 or 10 fibres in the presence of Fn or heparin, respectively, and error bars indicate s.d. Full size image Figure 4: Experimental validation of mechanosensitive binding of bacterial peptides to Fn fibres. ( a , b ) Strain-dependent binding of bacterial peptides B3C-Alexa488 and STAFF5C-Alexa488 to Cy5-labelled Fn fibres. The mean of the intensity ratios ( I B3C-488 / I Fn-Cy5 ) of relaxed fibres was set to 1 and the other values were scaled accordingly. All mean values (shown by black bar) are significantly different from each other with P <0.001 (unpaired two-tailed Student's t -test), except where noted. ( a ) Intensity ratio plot of Alexa488-labelled B3C to Cy5-labelled Fn fibres versus Fn fibre strain (see Fig. 3). Each experiment (shown as differently shaped and coloured data points) consisted of 30 fibres: 10 were relaxed ( ∼ 7% strain), 10 deposited only in a prestrained state (no mechanical manipulation of the silicone sheet, ∼ 140% strain [26] ) and 10 stretched ( ∼ 300 or ∼ 380% strain). ( b ) Intensity ratio plot of Alexa488-labelled STAFF5C to Cy5-labelled Fn fibres versus Fn fibre strain. Each experiment (shown as differently shaped and coloured data points) consisted of 40 fibres, including 20 relaxed ( ∼ 0 and ∼ 100% strain) and 20 stretched fibres ( ∼ 250 and ∼ 380% strain). Inhibition of strain-dependent binding of the bacterial peptide B3C-Alexa488 to Cy5-labelled Fn fibres in the presence (red bars) of ( c ) soluble Fn (300 μl mg −1 ) and ( d ) heparin (100 μl mg −1 ). The mean of the intensity ratio of relaxed fibres in the absence (blue bars) of soluble Fn or heparin was set to 1 and the remaining three values were scaled accordingly. All values are significantly different from each other (unpaired two-tailed Student's t -test) with P <0.0001, except where indicated. Values are means of intensity ratios of 20 or 10 fibres in the presence of Fn or heparin, respectively, and error bars indicate s.d. Full size image To demonstrate that mechanosensitivity is a more common feature of bacterial FnBPs, the experiment was repeated using a different peptide STAFF5, which is part of the fifth FnBR in the Fn-binding protein A (FnBPA) of S. aureus ( Fig. 1b,c ). The peptide STAFF5 binds to Fn using the same mechanism as B3C binding to Fn, but recognizes FnI 4,5 (ref. 29 ) close to the N-terminus of Fn. This peptide was also synthesized with an additional N-terminal cysteine residue that was used to conjugate Alexa Flour-488 dye (STAFF5C-488). As the mechanical strain increased, we observed a decrease in binding of STAFF5C-488 to Fn fibres, similar to our findings with B3C-488 ( Fig. 4b ). Mechanosensitive binding unaltered by heparin and soluble Fn The same N-terminal region of Fn to which most Gram-positive bacteria adhere also functions as a binding site for soluble Fn [30] and heparin [31] ( Fig. 1a ). High concentrations of soluble Fn are present in serum [32] , and heparin is frequently administered as a preoperative anticoagulant [33] . As both of these molecules might coregulate the binding of bacterial adhesins to Fn, we asked whether the presence of either one of the molecules might impact the force-regulated binding of bacterial FnBRs to fibrillar Fn. In the presence of physiological concentrations of soluble Fn (300 ìg ml −1 ), the binding of B3C to relaxed and stretched Fn fibres decreases by 40 or 60%, respectively, but is still strain dependent ( Fig. 4c ). Confirming the trend seen in Figure 4c , more bacterial peptide binds to relaxed than to stretched Fn fibres, which indicates that the peptide is sensitive to Fn fibre tension even in the presence of soluble Fn. The decrease in B3C binding to Fn fibres in the presence of soluble Fn could be attributed to either B3C binding to soluble Fn in solution without further interaction of this complex with fibrillar Fn, and/or soluble Fn binding to fibrillar Fn and partially blocking B3C binding to the fibres. Similar results were obtained for heparin, in which we observe a reduction in the binding of B3C to relaxed and stretched Fn fibres of 25 or 40%, respectively ( Fig. 4d ). This is in good agreement with an earlier study in which 100 μg ml −1 of heparin reduced bacterial adhesion to implant surfaces coated with Fn [34] . Our data indicate that both soluble Fn and heparin decrease the binding of bacterial adhesin to Fn fibres, but importantly the presence of either does not alter the mechanosensitivity of the binding of bacterial peptide to Fn fibres. Fn stretching causes structural mismatch of binding epitope To explore the underpinning mechanism by which tensile force exerting an effect on Fn fibres can disrupt bacterial-binding sites, we used SMD to simulate the stretching of FnI modules in complex with the bacterial peptide B3T (B3 truncated; Fig. 1c ). The nuclear magnetic resonance structure of the FnI 1-2 –B3T complex [15] (PDB 1O9A) was used as a starting structure for all simulations and hydrated in a box filled with explicit water molecules. The bacterial B3T peptide binds to both FnI modules by the antiparallel alignment of the two binding motifs on B3T with two distinct β-sheets formed by FnI 1 and FnI 2 . For SMD simulations, the solvated system was equilibrated for 2 ns before applying constant tensile force (defined as t =0 ns; Fig. 5a,b ). Three independent simulations were performed, each of which lasted for 7 ns. 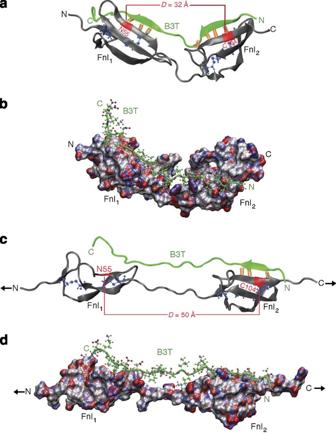Figure 5: SMD simulation of the FnI1,2–B3T complex illustrating the molecular mechanism of strain-induced unbinding. (a) Equilibrated structure at 0 ns. Backbone hydrogen bonds between Fn modules (grey) and the bacterial peptide (green) are shown as orange springs and the intramodular FnI disulphide bond forming cysteine residues are represented in blue. The distanceDis defined as the spacing between residues ASN55 on FnI1and CYS104 on FnI2, which are located at the centre of the respective module's binding site for B3T. (b) Molecular surface representation of the same complex, colour-coded according to charge (neutral: white or green, positive: red, negative: blue). (c) The complex at 5 ns after having applied a constant force (black arrows) of 400 pN to the Fn termini. (d) Molecular surface representation at 5 ns, colour-coded according to charge (neutral: white or green, positive: red, negative: blue). Figure 5: SMD simulation of the FnI 1,2 –B3T complex illustrating the molecular mechanism of strain-induced unbinding. ( a ) Equilibrated structure at 0 ns. Backbone hydrogen bonds between Fn modules (grey) and the bacterial peptide (green) are shown as orange springs and the intramodular FnI disulphide bond forming cysteine residues are represented in blue. The distance D is defined as the spacing between residues ASN55 on FnI 1 and CYS104 on FnI 2 , which are located at the centre of the respective module's binding site for B3T. ( b ) Molecular surface representation of the same complex, colour-coded according to charge (neutral: white or green, positive: red, negative: blue). ( c ) The complex at 5 ns after having applied a constant force (black arrows) of 400 pN to the Fn termini. ( d ) Molecular surface representation at 5 ns, colour-coded according to charge (neutral: white or green, positive: red, negative: blue). Full size image When stretching the FnI 1-2 modules with an external mechanical force of 400 pN applied to its terminal ends, the β-sheet formed between FnI 1 and B3T is destroyed after 2 ns of pulling ( Fig. 5c,d and Supplementary Movie 1 ). In addition, we observe that the distance between FnI 1 and FnI 2 increases (green curve in Fig. 6a ). This coincides with a decrease in the number of backbone hydrogen bonds formed between Fn and B3T (green curve in Fig. 6b ). While stretching the FnI 1-2 modules, the β-zipper motif formed with module FnI 1 was disrupted, whereas the backbone hydrogen bonds formed between FnI 2 and the bacterial peptide remained intact. In the second simulation, B3T detaches from FnI 2 but remains bound to FnI 1 (blue curves in Fig. 6a–c ). In the third simulation, the number of backbone hydrogen bonds decreases only slightly (red curve in Fig. 6b ). This is because the corresponding starting structure did not show a pronounced β-interaction between the carboxy (C)-terminus of B3T and FnI 1 and thus fewer bonds were broken when compared with the other two trajectories. We also observe a small increase in side-chain hydrogen bonds formed between Fn 1-2 and B3T (red curve in Fig. 6c ), which are able to form near the C-terminus of B3T. However, similar to the observations in the other two simulations, the distance between FnI 1 and FnI 2 increases (red curve in Fig. 6a ). 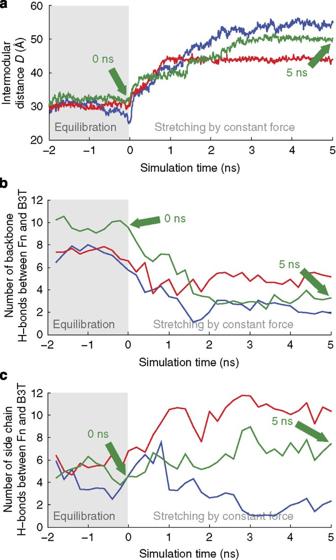Figure 6: Changes of intermodular distances and intermolecular hydrogen bonds formed between the FnI1–2–B3T complex as derived from steered molecular dynamic simulations. (a) Intermodular FnI1-FnI2distanceD(as defined inFig. 5a) plotted versus time for three independently conducted SMD simulations (different colour traces). A constant force of 400 pN is applied at time zero to stretch Fn. The green curves correspond to the simulation, the structures of which are presented inFigure 5, at the time points indicated by the green arrows. (b) Total number of backbone hydrogen bonds formed between FnI1-2and the peptide B3T versus time. (c) Total number of side-chain hydrogen bonds formed between FnI1–2and the peptide B3T versus time. Figure 6: Changes of intermodular distances and intermolecular hydrogen bonds formed between the FnI 1–2 –B3T complex as derived from steered molecular dynamic simulations. ( a ) Intermodular FnI 1 -FnI 2 distance D (as defined in Fig. 5a ) plotted versus time for three independently conducted SMD simulations (different colour traces). A constant force of 400 pN is applied at time zero to stretch Fn. The green curves correspond to the simulation, the structures of which are presented in Figure 5 , at the time points indicated by the green arrows. ( b ) Total number of backbone hydrogen bonds formed between FnI 1-2 and the peptide B3T versus time. ( c ) Total number of side-chain hydrogen bonds formed between FnI 1–2 and the peptide B3T versus time. Full size image In all three simulations, stretching Fn causes a structural mismatch leading to partial detachment of B3T from FnI 1-2 , where the formation of the tandem β-zipper is partially destroyed and reduced to a monomodular interaction between the bacterial peptide and one of the FnI modules. The number of side-chain hydrogen bonds fluctuates significantly and differs among simulations because of the large mobility of the bacterial peptide once it partially disconnects from the Fn fragment ( Fig. 6c ). However, in all our previous simulations of β-sheet motifs, we found that the major force-bearing interactions were defined by backbone and not by side-chain interactions [35] , [36] . 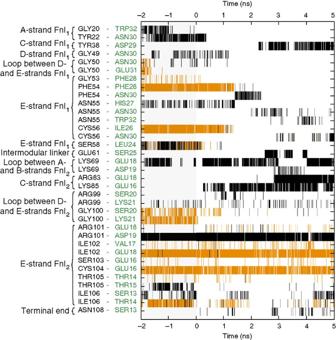Figure 7: Intermolecular backbone hydrogen and side chain hydrogen bond fluctuations within the FnI1–2–B3T complex plotted over simulation time. Residues on FnI1–2are listed in black text and residues on B3T in green. Only bonds that were present during 0.3 ns or longer are shown. Constant external force of 400 pN was applied starting at 0 ns. Backbone hydrogen bonds (orange) between FnI1and B3T are disrupted at∼1 ns (PHE54-PHE28 and CYS56-ILE26), whereas FnI2stays bound to B3T (ILE102-GLU18 and CYS104-GLU16). The total numbers of intermolecular hydrogen bonds for this simulation are plotted in the green curve inFigure 6, and the corresponding structures are displayed inFigure 5. Side chain hydrogen bonds are displayed in black. A detailed overview of both backbone and side-chain intermolecular hydrogen bonds observed in the first simulation can be found in Figure 7 . Our conclusions derived from this computational analysis agree with a very recent and independently conducted simulation [37] . Taken together, the insights gained from SMD simulations provide a high-resolution structural mechanism that shows how mechanical force pulling on Fn can affect the interaction between B3 and FnI 1-2 , thereby offering an explanation for the experimentally observed decrease in binding of the bacterial peptide to stretched Fn fibres. Figure 7: Intermolecular backbone hydrogen and side chain hydrogen bond fluctuations within the FnI 1–2 –B3T complex plotted over simulation time. Residues on FnI 1–2 are listed in black text and residues on B3T in green. Only bonds that were present during 0.3 ns or longer are shown. Constant external force of 400 pN was applied starting at 0 ns. Backbone hydrogen bonds (orange) between FnI 1 and B3T are disrupted at ∼ 1 ns (PHE54-PHE28 and CYS56-ILE26), whereas FnI 2 stays bound to B3T (ILE102-GLU18 and CYS104-GLU16). The total numbers of intermolecular hydrogen bonds for this simulation are plotted in the green curve in Figure 6 , and the corresponding structures are displayed in Figure 5 . Side chain hydrogen bonds are displayed in black. Full size image The finding that the specific binding of bacterial FnBR can be mechanically regulated ( Fig. 4 ) is to our knowledge the first experimental demonstration that mechanical forces functioning on ECM fibres can disrupt a cell-binding site. Various FnBPs that are intrinsically disordered in solution [38] engage up to five FnI modules ( Fig. 1 ) to form the tandem β-zipper that ensures specific binding. Insights into the structural mechanism that mediates the experimentally observed force-induced disruption of the bacterial adhesin interacting with FnI modules ( Figs 2 , 3 , 4 ) were obtained by SMD simulations ( Figs 5 , 6 , 7 ). Stretching of consecutive FnI modules bound to bacterial peptides increases the distance between the bacterial binding sites of Fn. This structural mismatch finally leads to the partial dissociation of the bacterial peptide from FnI modules ( Fig. 5c ), thus disrupting the multimodular interaction. Our results with the peptide STAFF5 derived from S. aureus ( Fig. 4b ) indicate that the structural unbinding mechanism described for the bacterial peptide B3 interacting with FnI 1-2 ( Fig. 5 ) might be more general. Experimental results from STAFF5 illustrate that mechanical forces functioning on Fn can also cause a strain-induced structural mismatch at FnI 4-5 , in which the two FnI modules are separated by a shorter linker chain than in FnI 1-2 . The FnI modules contain many other physiologically significant bindings sites, such as to heparin, collagen, tenascin and fibrin ( Fig. 1a ), which could also potentially be mechanoregulated. Soluble Fn and heparin are known to recognize the same N-terminal domain of Fn as the bacterial adhesins [11] ; therefore, we tested the binding of B3C to Fn fibres in the presence of soluble Fn and heparin. The binding of bacterial peptide to Fn fibres is significantly reduced in both instances ( Fig. 4c,d ), which correlates well with previous studies that show inhibition of FnBP-mediated bacterial adhesion to Fn-coated surfaces [34] , [39] . The question arises whether the observed inhibitory effects would also be relevant in vivo , as the K d of B3C (a part of an FnBR) to Fn fragments is about 1 μM [15] , whereas complete FnBR can bind to Fn with nanomolar affinity [10] because of the multimodularity of the interaction. However, it is important to note that the affinities were measured to Fn fragments in solution, and not to (full-length) fibrillar Fn. Furthermore, in the case of heparin, evidence suggests that the binding site is located on loop regions and not on the β-strands of the FnI modules [31] , meaning that heparin and bacterial FnBRs do not necessarily compete for the same epitope on Fn. Hence, it is possible that heparin sterically hinders the binding of bacterial peptides to Fn. Regardless of the degree of the observed inhibition, our results indicate that the mechanosensitivity of the FnBP–Fn interaction remains unaltered even in the presence of soluble Fn and heparin at physiological concentrations. Notably, the force-regulated mechanism discovered here is distinctly different from the catch-bond mechanism that some bacteria have evolved to adhere to surfaces under fluid flow [40] . In the case of E. coli adhesion (type 1 fimbriae adhere to mannose), force regulation is achieved by fluid shear stress pulling on a ligand that sits in a binding pocket, thereby activating the long-lived catch-bond state. In contrast, the binding of bacterial FnBR is weakened by stretching Fn, for example, by cell-generated forces. In this case, the force exerts an effect along the Fn fibre axis and destroys the structural match between the receptor and ligand, thereby inhibiting binding even in situations where no force directly pulls on the bacterial adhesin. Can cells sufficiently stretch ECM fibres to activate the FnI mechanical adhesion switch and thus downregulate the binding of bacterial adhesins? Quantifying this in cell culture is difficult because of the high density of spatially colocalized conformations of differently stretched Fn, as well as the temporal variations in fibre tension [24] , [27] . It is important to recognize that the Fn strains in our binding assays are within the regime of strains displayed by Fn matrix in cell culture, as shown by fluorescence resonance energy transfer measurements: A considerable fraction of Fn fibres are known to be stretched more than threefold by cells in two-dimensional and three-dimensional cell cultures [27] , [41] depending on the contractility of the cells and the physiological state of ECM. The observed decrease in binding occurs at Fn fibril strains of 300% or more, whereas in SMD simulations the unbinding of B3T occurs at FnI 1-2 strains of about 50%. This is due to the different mechanical stabilities of the more than 50 different modules per dimeric Fn (types I, II and III). Besides increasing the intermodular distances of FnI modules, the mechanical force pulling on Fn fibre also stretches out the other modules and triggers the unfolding of FnIII modules [24] . As the force needed to activate the increase in the intermodular distance between FnI modules is roughly comparable to that of unfolding the first FnIII modules [35] , [42] , the increase in the intermodular distances between FnI modules only partially contributes to the total strain of a Fn fibre. Because of the intrinsic limits for how long all-atom simulations can be run, forces used in SMD simulations are typically higher than those physiologically observed [43] . It is important to note though that it is not the direct correlation with force but the force-induced mechanical strain that defines the switch in the structure–function relationship of stretched proteins. The key motivation for conducting SMD simulations is to identify the force-stabilized structural intermediate states. Several structural mechanisms initially deduced from SMD for other protein systems have been experimentally validated. This includes studies showing the derivation of a first-structural model showing how catch-bond-forming bacterial adhesins work [40] , [44] , structural predictions proposing a mechanism that elucidates how stretching talin causes the exposure of vinculin-binding sites [45] , [46] , elucidating the structural mechanism of how titin kinase is force activated [47] and recent efforts to engineer proteins with enhanced mechanical properties [48] . Taken together, all these observations indicate that our assay using manually deposited Fn fibres provides physiologically relevant insights, and that cell-generated forces are sufficiently high to deactivate the specific binding of bacterial adhesins. However, it should be noted that mechanoregulation of the specific interactions between bacterial FnBP and Fn fibres might be masked since the long protrusions that define bacterial adhesins comprise many other specific and nonspecific binding sites. Each of these epitopes could have a different or non-existent mechanosensitivity. Furthermore, the stretching of Fn fibres gradually exposes hydrophobic amino acids because of the loss of secondary structure, thus additionally promoting nonspecific adhesion [25] . Many prokaryotic and eukaryotic cell adhesins have evolved polyvalent structural motifs in order to interact with their target host proteins ( Fig. 1a ). For instance, integrins α5β1 and αIIaβ3 both recognize not just the RGD (arginine-glycine-aspartic acid)–loop on FnIII 10 but also the adjacent synergy site on FnIII 9 [49] , thus exploiting a bivalent binding strategy to Fn tandem modules to enhance interaction. Interestingly, phylogenetically distinct bacteria use similar motifs to bind to Fn but differ in the number of binding repeats. Multivalent interactions in general extend the lifetime of molecular interactions [50] . How pathogens exploit multivalency in order to colonize highly specialized niches by optimizing their adhesins is poorly understood. Our data provide the first hints that this divergence might equip bacteria with a sensory tool to differentially probe ECM tension. It is of paramount importance to understand how bacteria evolved their adhesins to optimize their strategies for host invasion and infection. This first demonstration of a mechanoregulated binding site raises intriguing questions whether bacteria can distinguish healthy tissue from wound sites by sensing matrix tension exerting an effect on Fn fibres. At wound sites and areas of inflammation, the ECM fibres are physically or proteolytically cleaved, which should lead to their relaxation. Injured or diseased tissues might thus present Fn in different physical states, and we speculate that this could regulate early adhesion events. The finding that the specific binding of adhesins might be regulated by the tension of ECM fibres provides a unique and new perspective on how the mechanobiology of ECM might regulate early bacterial adhesion and the subsequent course of infection. Isolation of Fn and protein labelling Fn was isolated from human plasma (Zürcher Blutspendedienst SRK) using gelatin-sepharose chromatography based on established methods [51] . Experiments were approved and authorized by the SwissFederal Office for the Environment and Swiss Federal Coordination Center for Biotechnology (notification number A080170). Briefly, 2 mM phenylmethylsulphonyl fluoride and 10 mM EDTA were added to human plasma and spun at 15,000 g for 40 min. Plasma was first passed over the gelatin Sepharose 4B column (Pharmacia) and subsequently the flow-through passed over the Sepharose 4B column (Sigma-Aldrich). The gelatin column was washed with 2 mM phenylmethylsulphonyl fluoride and 10 mM EDTA in PBS. Wash completion was verified when the 280 nm absorbance of the flow-through was <0.05. The gelatin column was washed with 1 M NaCl, 1 M urea, and finally Fn was eluted from the column with 6 M urea. Purity was approximated by silver stain and western blot. Isolated Fn was stored at −80 °C in 6 M urea until usage. The buried cysteines within modules FnIII 7 and FnIII 15 of each Fn dimer were site-specifically labelled with Cy5-maleamide (647 nm; Molecular Probes, Invitrogen) following established protocols [24] , [27] . Briefly, isolated plasma Fn at about 5 g l −1 in PBS was denatured in an equal volume of 8 M GdnHCl and incubated for 1 h with a 20-fold molar excess of Cy5-maleimide at room temperature. The labelled Fn was then separated from the free dye by size exclusion chromatography (PD-10 Sephadex, Amersham) into PBS. The labelling ratio of Cy5 per Fn dimer was determined by measuring the absorbance of Fn-Cy5 at 280 and 647 nm and using published extinction coefficients for the fluorophore and Fn. The labelled Fn was stored at −20°C until needed and used within 2 days of thawing. Before use, labelled and unlabelled Fn aliquots were centrifuged at 10,000 g for 10 min to remove aggregates. The bacterial B3C moiety from S. dysgalactiae and STAFF5C from S. aureus were synthesized (Genscript Corporation) with a terminal cysteine for photolabelling (peptide sequences are given in Fig. 1c ). A 200 μg ml −1 solution of each peptide was labelled with Alexa Fluor 488 (Molecular Probes, Invitrogen) as described above and stored at −20 °C until needed. Fn fibre assembly and deposition on stretchable silicone sheets Fn fibres were pulled from a concentrated droplet of Fn solution and deposited on silicone sheets (Speciality Manufacturing). The silicone sheets were mounted and stretched in a one-dimensional strain device as previously described ( Fig. 2b ) [27] . Briefly, 0.25-mm-thick silicone sheets were cut into 5×1.7 cm rectangles and a 300 μg ml −1 Fn solution (5% Fn-Cy5, 95% unlabelled) was deposited as a small drop on the sheet. With the aid of a pipette tip, Fn Fibres were drawn by hand out of the droplet and deposited ( Fig. 2a ). The samples were rinsed and kept hydrated with PBS. The fibres were either deposited in parallel or perpendicular to the strain axis. The fibres are deposited on a prestrained sheet (150% strain), which is relaxed in the x axis and results in stretching of the sheet in a transverse direction when using a one-dimensional straining device. Fibre strain was calculated from the externally adjusted strain of the silicone sheet as previously described [24] . The intensity ratios of the samples were measured with confocal microscopy as described below. Assay to probe the binding of bacterial adhesins to fibrillar Fn To quantify bacterial peptide binding to fibrillar Fn, samples of manually deposited fibres were prepared and incubated with 0.1 M iodoacetamide to alkylate any free cysteine that might get exposed by fibre stretching [25] , [26] , [27] and could potentially react with free Alexa-488 maleimide dye. This was followed by incubation with 4% bovine serum albumin for 30 min to block nonspecific binding. Finally, after rinsing with PBS, the samples were incubated with B3C-Alexa488 or STAFF5C-Alexa488 for 30 min. The sample was finally rinsed with PBS (3×) and imaged under hydrated conditions (that is, immersed in PBS) at room temperature. Confocal microscopy All confocal images were acquired with an Olympus FV1000 confocal microscope (Olympus) with a water immersion 0.9 NA ×40 objective. Emitted light from the sample, as well as differential interference contrast images, were detected with two photomultiplier tubes. Images were acquired at 512 × 512 pixel resolution for a 318 by 318 μm field of view. Acquisition parameters including laser transmissivity, pixel dwell time and pinhole size were adjusted to prevent photobleaching while maximizing detection sensitivity. Photomultiplier tube gains were kept constant during measurements within an experiment. Image analysis Confocal images were analysed using MatLab (MathWorks) and ImageJ. The dark current values were subtracted and the images were scanned and all pixels above a certain threshold were considered as being part of the fibre (to avoid inclusion of intensity peaks of the background). The ratios presented in Figure 3 were taken by dividing the mean of the intensity at 488 nm (that is, the intensity stemming from the Alexa488-labelled bacterial peptide) by the mean of the intensity at 633 nm (that is, the intensity stemming from the Cy5-labelled Fn fibre). All analysed images have a resolution of 512 by 512 pixels. Computer simulations Simulations were performed using the open-source molecular dynamics software NAMD and the CHARMM27 force field [52] . The program VMD was used as a visualization tool [53] . Long-range electrostatic forces were calculated with the particle mesh Ewald summation with a grid size of <1 Å. Van der Waals interactions were simulated using a switching function starting at 10 Å and a cutoff of 12 Å. We used three nuclear magnetic resonance structures of the FnI 1,2 –B3 complex from S. dysgalactiae , which were obtained from PDB (accession code 1O9A ) [15] . For every simulation, the structure was placed in an explicit TIP3P water box [54] and ions were added to obtain an electrically neutral system with a physiological salt concentration of 0.15 M. The water box was designed to have 15 Å padding along two axes and 40 Å along the third direction, so as to give the molecule enough space while elongating. The system was then minimized for 2,000 steps while keeping all atoms of the protein fixed. Another 2,000 steps were performed keeping only the backbone atoms of the protein fixed. The next 2,000 steps were performed without fixation of any atoms. This was followed by thermalizing the system, wherein the temperature was raised by 1 K every 100 steps up to 310 K. Thereafter, the system was equilibrated for 2 ns (with an integration time step of 1 fs) using the Berendsen method for keeping both temperature and pressure ( P =1 atm) constant [55] . A constant force of 400 pN was then applied to the two terminal C-α atoms of the protein backbone. The force vectors were pointing in opposite directions along the elongation of the water box. During the first ∼ 100 ps of pulling, the protein aligned to the force direction. Hydrogen bonds were analysed using a distance cutoff of 3.51 Å and an angle cutoff of 30.1°. All simulations were performed on 128 nodes of a Cray XT-3 cluster located at the Swiss National Supercomputing Centre (CSCS). How to cite this article: Chabria M. et al . Stretching fibronectin fibres disrupts binding of bacterial adhesins by physically destroying an epitope. Nat. Commun. 1:135 doi: 10.1038/ncomms1135 (2010).